Cryo-EM structures of lipopolysaccharide transporter LptB2FGC in lipopolysaccharide or AMP-PNP-bound states reveal its transport mechanism Lipopolysaccharides (LPS) of Gram-negative bacteria are critical for the defence against cytotoxic substances and must be transported from the inner membrane (IM) to the outer membrane (OM) through a bridge formed by seven membrane proteins (LptBFGCADE). The IM component LptB 2 FG powers the process through a yet unclarified mechanism. Here we report three high-resolution cryo-EM structures of LptB 2 FG alone and complexed with LptC (LptB 2 FGC), trapped in either the LPS- or AMP-PNP-bound state. The structures reveal conformational changes between these states and substrate binding with or without LptC. We identify two functional transmembrane arginine-containing loops interacting with the bound AMP-PNP and elucidate allosteric communications between the domains. AMP-PNP binding induces an inward rotation and shift of the transmembrane helices of LptFG and LptC to tighten the cavity, with the closure of two lateral gates, to eventually expel LPS into the bridge. Functional assays reveal the functionality of the LptF and LptG periplasmic domains. Our findings shed light on the LPS transport mechanism. Antibiotic resistance of Gram-negative bacteria has become one of the greatest threats to global health [1] . The asymmetric outer membrane (OM) of Gram-negative bacteria has a crucial role in defending against extracellular cytotoxic molecules such as antibiotics [2] . Lipopolysaccharide (LPS) is the main component of the OM, and its importance is not only in maintaining the OM structure, shielding from harmful molecules but also inducing host inflammatory immune responses causing disease-like sepsis [3] , [4] , [5] . Compromised OM integrity reduces virulence of pathogenic bacterial species and increases their sensitivity to antimicrobial agents [6] . LPS is a large glycolipid consisting of lipid A, core oligosaccharide and O-antigen [5] , [7] , [8] . Components of LPS are synthesised in bacterial cytoplasm and then transported onto the periplasmic side of the inner membrane (IM), from where mature LPS is assembled and transported to the OM [9] , [10] , [11] , [12] . Seven LPS transport proteins (LptBFGCADE) form a trans -envelope bridge for LPS transport from the IM to the OM across the aqueous periplasm [13] , [14] , [15] , [16] , [17] , [18] , [19] , [20] , [21] , [22] , [23] , [24] , [25] (Fig. 1a ), which is a potential target for novel antimicrobial drugs [26] , [27] , [28] , [29] . The IM component LptB 2 FG comprises an ATP-binding cassette (ABC) transporter, which powers the transport of LPS across the bridge. The cytoplasmic LptB dimer binds and hydrolyses ATP and the transmembrane (TM) domains of LptF and LptG create a cavity to accommodate LPS (Fig. 1a ). Unlike other canonical bacterial ABC transporters, which translocate substrate across the IM, LptB 2 FG acts by extracting LPS from the periplasmic side of the IM and delivering it to the periplasmic domain of the IM protein LptC [18] , [30] , [31] , [32] , [33] , [34] . LptC, which consists of a TM helix and a jellyroll-like periplasmic domain, forms a stable complex with LptB 2 FG to receive LPS and deliver it to the periplasmic protein LptA in the bridge [32] , [35] (Fig. 1a ). Fig. 1 Architecture of LPS-bound sf LptB 2 FG complex. a A scheme of seven lipopolysaccharide transport proteins form a trans -envelope bridge to transport LPS from the IM to the OM. b Left panel: a cross-sectional view of cryo-EM map of LPS-bound sf LptB 2 FG; Right panel: a closed view of LPS. A clear density for LPS is shown in blue mesh and LPS is shown in stick. LptF, LptG and the two LptB molecules are presented in cartoon and coloured in cyan, purple, green and yellow, respectively. c Cartoon representation of LPS-bound sf LptB 2 FG. An LPS molecule, shown in spheres, is located in the upper cavity of the transmembrane channel. d Rotation of 180° along the y -axis relative to c Full size image To understand the mechanisms of how LptB 2 FGC recognises and acts to transport LPS, we obtained high-resolution cryo-electron microscopy (cryo-EM) structures of LptB 2 FGC complexed with substrate LPS or ATP analogue β-γ-imidoadenosine 5′-triphosphate (AMP-PNP). We also obtained cryo-EM structure of LptB 2 FG complexed with LPS to compare the conformational changes with and without the presence of LptC. Two recent studies reported LptB 2 FGC structures: the work of Owens et al. [36] is an X-ray crystallographic study of Vibrio cholerae and Enterobacter cloacae LptB 2 FGC in detergent micelles and the work of Li et al. [37] is a cryo-EM study of Escherichia coli LptB 2 FGC in lipid nano-discs with and without ADP-vanadate. Although LptB 2 FGC complex structures have been studied, due to partial occupancy or low resolutions in the substrate or nucleotide-binding pockets the two papers show no atomic evidence to determine LPS recognition in LptB 2 FGC complex or nucleotide-binding-induced transport mechanism [36] , [37] . By contrast, our high-resolution cryo-EM structures reveal atomic details in the LPS-binding and ATP-binding cavities, and mutagenic assays allowed us further to identify functional residues in the TM cavity and two periplasmic domains of LptF and LptG involved in LPS recognition and transport process including two essential arginine residues LptF R292 and LptG R301 in the cytoplasmic loop 2 of LptF or LptG. Conformational changes and molecular shifts between domains upon nucleotide binding reveal working mechanism of the transporter. The ATPase activities of purified LptB 2 FG and LptB 2 FGC LptB 2 FG and LptB 2 FGC from Shigella flexneri ( sf LptB 2 FG and sf LptB 2 FGC) were cloned, overexpressed, solubilised in n -dodecyl-β- d -maltopyranoside (DDM), and purified in Lauryl maltose-neopentyl glycol (LMNG) (Supplementary Fig. 1a, b ). The ATPase activity of sf LptB 2 FG and sf LptB 2 FGC were measured (Supplementary Fig. 1c, d ). Comparing to sf LptB 2 FG, the ATPase activity of sf LptB 2 FGC is about 50% less under the same conditions, confirming the reported regulatory role of LptC to the LptB 2 FG transporter [36] , [37] . The ATP non-hydrolysable analogue AMP-PNP significantly inhibits the ATPase activity of sf LptB 2 FGC, which was used to mimic and lock an ATP-bound state of sf LptB 2 FGC. Cryo-EM structure of LptB 2 FG in LPS-bound state Our previous published crystal structure of LptB 2 FG from Klebsiella pneumonia ( kp LptB 2 FG) did not identify the bound LPS molecule due to low resolution and low occupancy, although an extra electron density was found in the cavity [38] . In this study, we used cryo-EM to resolve an LPS-bound structure of sf LptB 2 FG at overall 3.7 Å resolution with TM domain at 3.2 Å resolution (Supplementary Figs. 2 and 3 ). The cryo-EM maps of sf LptB 2 FG show clear side chain densities in the nucleotide-binding domains (NBDs) and the two transmembrane domains (TMDs), allowing us to unambiguously fit models of NBDs and TMDs of LptB 2 FG (Fig. 1b ). LptB 2 constitutes the cytoplasmic NBD dimer and the six TM helices of LptF and LptG (F_TM1-TM6 and G_TM1-TM6) constitute two TMDs that are arranged to form a central cavity with two surface gaps between TM1F and TM5G and TM1G and TM5F termed as lateral gates (Fig. 1c, d ). The densities for the periplasmic domains of LptF and LptG are at low resolution but are clearly visible (Fig. 1b and Supplementary Fig. 3 ). Each TMD has two cytoplasmic loops: loop 1 links the TM2 and TM3 helices through the coupling helix and loop 2 links the TM4 and TM5 helices of LptF and LptG (Fig. 1c, d ). The cryo-EM structure reveals a clear LPS density in the central cavity (Fig. 1b ), showing all six acyl tails, glucosamine disaccharide phosphorylated at 1′ and 4′ positions, and the inner core oligosaccharide. The LPS molecule trapped is a natural substrate of sf LptB 2 FG that was overexpressed in the E. coli C43(DE3) strain. The acyl tails of LPS are drooped and perpendicular to the IM plane in the upper cavity and the inner core positioned above in the periplasmic space (Fig. 1b–d ). In the cavity, hydrophobic residues I25, F26, L62, L66, L70 and M303 of LptF and L26, I33, I66, F67, I313, F317 and Y320 of LptG interact with the LPS acyl tails via van der Waals interactions. Charged residues K34, K62, R133 and R136 of LptG and R33 of LptF form salt bonds with the 1′-phosphate group of LPS, while K40 of LptG and K317 of LptF form salt bonds with the 4′-phosphate group of LPS. D37 of LptG interacts with the glucosamine disaccharide of lipid A. K322, R263 and Q248 of LptF and K41 of LptG interact with the inner core oligosaccharide (Fig. 2a, b ). Previously, we reported that mutants of the hydrophobic residues F26D and L62D of LptF in the cavity severely impaired cell viability [38] . Here we carried out functional assay amongst those conserved charged and hydrophobic residues of LptG and found that K34E, R136E, R133E/K136E, Y257E/Y271E and F67E/Y320E are lethal (Fig. 2c, d and Supplementary Fig. 4 ). Interestingly, alanine substitution K34A and R136A and single mutant Y257A, Y271A, F67A and Y320A are normal (Supplementary Fig. 4 ). The positively charged K34 and R136 and the hydrophobic F67 and Y320 are located in the upper cavity in proximity to the negatively charged phosphate group and the hydrophobic acyl chains of the bound LPS, respectively. These results suggest that K34, R136, F67 and Y320 are important to LPS binding by forming ionic bonds and hydrophobic interactions, respectively, which can be compensated by each other if one of these interactions is lost as no effect was seen in the single alanine mutations. However, introducing negatively charged substitution would result repulsive force to destabilise the ionic bond thus affecting the functionality of the complex. On the other hand, Y257 and Y271 are located outside the cavity at the interface between the TM and the periplasmic domain of LptG (Fig. 2a–d and Supplementary Fig. 4 ). Although not interacting with LPS, double mutant Y257E/Y271E abolishes the functionality of the transporter causing cell death, suggesting that their roles are not in LPS recognition but may be involved in later stage of LPS transport to the bridge. In contrast, mutation of residues located in the lower cavity of LptG such as K13E/R86E showed no effect on cell viability, suggesting that the lower cavity is not involved in LPS binding (Supplementary Fig. 4 ). The high resolution within the LPS-binding cavity of the structure allowed us to visualise that these residues interact with the trapped LPS, supporting the results of the functional assays carried out here and reported before [39] , [40] . Fig. 2 s f LptB 2 FG recognition of LPS. a Residues of LptF and LptG from the cavity that interact with LPS. LPS is shown in sphere and grey, whereas residues of LptF and LptG are shown in cyan and magenta, respectively. b 180° rotation of a along y -axis. c Functional assays of LptG residues. Mutants R136E, F67E/Y320E, Y257E/Y271E and K34E are lethal, whereas mutants R133E, K62E and L26E/M70E do not affect the bacterial growth. d Expression level of LptF and LptG of the mutants. The western blot showed that the mutant protein expression levels are similar to that of the wild type. Source data for panel d are provided as a Source Data file Full size image Cryo-EM structures of LptB 2 FGC in LPS-bound state The cryo-EM structure of sf LptB 2 FGC was determined to 3.1 Å resolution (Fig. 3a–d and Supplementary Figs. 5 and 6 ). The map shows clear densities of the TM helix of LptC located at one lateral gate between TM1G and TM5F, which is consistent to the published structures [36] , [37] (Fig. 3a and Supplementary Fig. 6 ). However, due to possible flexibility, we are unable to see clear density for the periplasmic domain of LptC (Fig. 3a and Supplementary Fig. 6 ). This was also the case in the recent reported cryo-EM structure of LptB 2 FGC, where most of particles collected do not show density for the periplasmic domain of LptC [37] , whereas on the other hand the reported crystal structure of LptB 2 FGC was able to show clear periplasmic domains [36] . In our structure, residues M1, R5, I9, L12, V16, M19 and N23 from the TM helix of LptC interact with residues Q293, L300, L305, L304, L307, L311 and T314 from the TM5 of LptF, respectively. In contrast, only G21 from the TM helix of LptC interacts with V36 of TM1 of LptG (Fig. 3b ). Comparing to the sf LptB 2 FG LPS-bound structure, the presence of the TM helix of LptC makes the lateral gate TM1G/TM5F of sf LptB 2 FGC structure much widely opened, along with the neighbouring TM2 and TM3 of LptG and TM4 and TM6 of LptF moved outward, resulting an enlarged central cavity (Fig. 3e, f ). In contrast to the two recent publications [36] , [37] , a density for LPS is identified in the cavity of sf LptB 2 FGC with all features visible as in the sf LptB 2 FG structure except the inner core of the LPS (Fig. 3a–d ). Interestingly, the LPS molecule trapped in the cavity of sf LptB 2 FGC is about 7.3 Å away from that of sf LptB 2 FG structure referring to the position of the 1′-phosphate group (Fig. 3e, f ). The LPS molecule in the sf LptB 2 FGC structure positions in proximity to LptG with kinked acyl tails rather than drooped as seen in the sf LptB 2 FG structure (Fig. 3b–d and Supplementary Fig. 6 ). In the cavity of sf LptB 2 FGC, we can also see that hydrophobic residues L17 and M24 from the TM helix of LptC interact with the bound LPS (Supplementary Fig. 7 ), suggesting that the TM helix of LptC is also involved in LPS recognition. The number of residues from the TM helices of LptF and LptG that have been shown to interact with LPS in the enlarged cavity of sf LptB 2 FGC are greatly reduced compared to the structure of sf LptB 2 FG (Fig. 3a, b and Supplementary Fig. 7 ). The weaker LPS binding in the cavity of sf LptB 2 FGC suggests an energy regulatory role of LptC in the transporter. The presence of LptC in the structure enlarges the gap at one lateral gate TM1G/TM5F, which makes one to speculate that LPS may enter the cavity via this lateral gate. We can visualise a detergent molecule (LMNG) trapped at this lateral gate. However, we found one acyl chain of the trapped LPS stuck at the opposite lateral gate TM1F/TM5G (Supplementary Fig. 8 ), suggesting that hydrophobic molecules to enter through these lateral gates is also possible. Fig. 3 Cryo-EM structure of LPS-bound sf LptB 2 FGC. a Cryo-EM map of LPS-bound sf LptB 2 FGC. The colour scheme is the same as in Fig. 1 . LptC is coloured in blue. b A close view of LPS. Lipid A of LPS is visible in the complex and LptC transmembrane helix is at the lateral gate TM1G/TM5F. LPS is shown in spheres. c Cartoon representation of LPS-bound sf LptB 2 FGC. d Rotation of 180° along the y -axis relative to c . e Periplasmic view of LPS-bound sf LptB 2 FG, where LPS is closed to the LptF side. f Periplasmic view of LPS-bound sfLptB 2 FGC. LPS is closed to the LptG side Full size image Cryo-EM structures of LptB 2 FGC in AMP-PNP-bound state To obtain a nucleotide-bound structure, we incubated the purified protein sf LptB 2 FGC with the non-hydrolysable ATP analogue AMP-PNP. Unlike the sf LptB 2 FGC LPS-bound structure, LptC is moved away from the lateral gate TM1G/TM5F so that the TM helix became invisible in the complex structure despite of the high resolution of 3.5 Å showing near atomic details in the cavity of the transporter (Fig. 4a–d , and Supplementary Figs. 9 and 10 ). Densities for the periplasmic domains of LptF and LptG are observed at low resolution but the periplasmic domain of LptC is unable to be visualised, which is also the case in the recently reported ADP-vanadate complexed LptB 2 FGC structure [37] (Supplementary Fig. 10 ). Superimposition of the two cryo-EM structures of sf LptB 2 FGC LPS-bound and sf LptB 2 FGC AMP-PNP-bound showed two different conformations with a root mean square deviation (RMSD) of 3.21 Å over 589 aligned Cα atoms (Fig. 5a, b ), representing two different states of the transporter. Fig. 4 Structure of AMP-PNP-bound sf LptB 2 FGC. a Cryo-EM map of AMP-PNP-bound sf LptB 2 FGC. The LptC density is not observed. Density of AMP-PNP is shown in blue mesh and AMP-PNP is shown in stick. The colour scheme is the same as Fig. 1 . b Rotation of 180° along the y -axis relative to a . c Cartoon representation of AMP-PNP-bound sf LptB 2 FGC. AMP-PNP is shown in spheres with carbon colour in green or yellow. DDM is shown in sphere with carbon in grey. d Rotation of 180° along y -axis relative to c . The DDM molecule is trapped in the lateral gate TM1F/TM5G Full size image Fig. 5 Superimpositions of AMP-PNP and LPS-bound sf LptB 2 FGC structures. a AMP-PNP binding induces the conformational changes of LptB (NDBs). The helical domains of the dimeric LptB (AMP-PNP-bound sf LptB 2 FGC) showed a rotational shift of ~12 Å in the anti-clockwise direction from the nucleotide-free state of dimeric LptB (LPS-bound sf LptB 2 FGC). The LPS-bound sf LptB 2 FGC is coloured in the same as Fig. 1 . The AMP-PNP-bound sf LptB 2 FGC is coloured in marine blue and AMP-PNP shows as spheres. b A top view of superimposed transmembrane helices of LPS-bound sf LptB 2 FGC and AMP-PNP-bound sf LptB 2 FGC complex. AMP-PNP binding induces the TM helices of AMP-PNP-bound sf LptB 2 FGC to rotate in the anti-clockwise direction with the largest shift of ~10 Å from the nucleotide-free state (LPS-bound sf LptB 2 FGC) towards the central channel. c Slab view of surface representation of cavity of LPS-bound sf LptB 2 FG. The cavity is in an outward open conformation. d Slab view of cavity of LPS-bound sf LptB 2 FGC. The cavity is in an outward open conformation. The transmembrane helix of LptC is located at the lateral gate TM1G/TM5F, enlarging the cavity. The neck of the cavity is widely open. e Slab view of cavity of AMP-PNP-bound sf LptB 2 FGC. The cavity is closed, which is induced by AMP-PNP binding Full size image In our structures, the sf LptB 2 FG and sf LptB 2 FGC process an open cavity to accommodate LPS (Fig. 5c, d ), while the sf LptB 2 FGC AMP-PNP-bound structure adopts a closed central cavity with a closed dimeric conformation of LptB (Fig. 5e ). The NBDs (LptB 2 ) of our sf LptB 2 FGC AMP-PNP-bound structure is similar to that of the ATP-bound E. coli LptB dimer (PBD: 4QC2) with a RMSD of 0.91 Å over 457 aligned Cα atoms [41] , particularly their bound nucleotides and the binding elements of LptB match well (Supplementary Fig. 11 ). A superimposition of the sf LptB 2 FGC AMP-PNP-bound structure and the nucleotide-free sf LptB 2 FGC LPS-bound structure shows that the binding of AMP-PNP causes an anti-clockwise rotation in the C terminal helical domains of LptB 2 towards the dimerisation interface (Fig. 5a ). The AMP-PNP binding also induces the conformational changes of TM1–5 of LptF and TM1–5 of LptG to rotate anti-clockwise toward the centre of the cavity (Fig. 5b ), resulting in a closed central cavity with a widely opened neck at the periplasmic side of the cavity (Fig. 5e ). No densities of LPS in this closed cavity was observed, suggesting a post-exporting state of LPS. Two lateral gates TM1F/TM5G and TM1G/TM5F shift into a closed conformation with their respective TM1 and TM5 helices oriented parallel to each other in close proximity, a ‘ cis ’ conformation (Supplementary Fig. 8 ). In this structure, a detergent molecule (DDM) is trapped at the lateral gate TM1F/TM5G, with hydrophobic tails trapped in the cavity while its hydrophilic head extends into the periplasm. The hydrophobic residues L16, I18, I21, I25 and M74 of LptF, and V309, V310, I313, L74, L78 and M25 of LptG in the lumen of the cavity interact with the detergent molecule (Supplementary Fig. 8 ). Some of these hydrophobic residues (e.g. residues I25 of LptF, residues L74 and I313 of LptG) are also involved in LPS binding (Fig. 2a, b ). As a result, the state of the trapped detergent molecule in the lateral gate may suggest the way that LPS enters the cavity of sf LptB 2 FGC. LptF R292 and LptG R301 interact with the bound AMP-PNP The sf LptB 2 FGC AMP-PNP-bound structure shows a closed dimeric conformation of LptB with clear densities for two bound AMP-PNP molecules in the ATP-binding sites at the interface of the NBDs (LptB dimer) (Fig. 4a–d ). Several residues are involved in the AMP-PNP binding site, including Y13, T44, T43, Q85, K42, E163, H195 and N38 from one LptB of the NBDs and E142, L138 and S139 from another LptB of the NBDs (Fig. 6a, b ). Some of these residues have been tested by the functional assays in previously published studies showing that mutations of these residues impaired bacterial cell viability [31] , [41] . In addition to the residues of LptB 2 , we also found that two arginine residues LptF_R292 and LptG_R301 on the cytoplasmic loop 2 of LptF and LptG extended ~9.8 and ~9.1 Å, respectively, toward the NBDs to interact with the bound AMP-PNP molecules (Fig. 6c, d ). To test whether these arginine residues are critical for the functionality of sf LptB 2 FGC, we made two single mutants LptF R292A and LptG R301A and tested cell viability and ATPase activity of the transporter. Interestingly these mutations showed no impact on the ATPase activity of the complex (Supplementary Fig. 1 ) but caused cell death in the functional assays (Fig. 6e, f ), suggesting that LptF R292 and LptG R301 residues are essential for LPS transporting but not ATP hydrolysing function of the transporter. As these loops connect TM helices that constitute the central cavity and lateral gates, we speculate that these cytoplasmic R292 and R301 containing loops probably act similarly to the coupling helices (cytoplasmic loop 1), which trigger conformational changes in the TMDs by allowing allosteric communication between the NBDs and TMDs of LptB 2 FGC upon nucleotide binding [33] . Fig. 6 R292 of LptF and R301 of LptG are involved in AMP-PNP binding. a A close view of AMP-PNP binding residues with dimeric LptB and R292 of LptF. b A close view of AMP-PNP binding residues with dimeric LptB and R301 of LptG. AMP-PNP molecules are shown in stick, and the cryo-EM map for AMP-PNP are shown in red mesh. c The two cryo-EM structures are superimposed. The arginine residue R292 located on the cytoplasmic loop 2 of LptF shifts around 9.8 Å to interact with AMP-PNP. d The arginine R301 located on the cytoplasmic loop 2 of LptG shifts around 9.1 Å to interact with the AMP-PNP. AMP-PNP molecules are shown in stick, the colour scheme of sf LptB 2 FGC AMP-PNP bound is the same as in Fig. 4 , and sf LptB 2 FG LPS bound is coloured in blue. e Functional assays of the single mutants R292 of LptF and R301 of LptG. NR1113 cells were transformed with empty vector (pTRC99a_Kan, the negative control) or the vector encoding LptB 2 F(Flag)G(Myc)C (the positive control). f Detection of protein expression levels of mutants by western blotting. Empty vector (pTRC99a_Kan, the negative control) or the vector encoding LptB 2 F(Flag)G(Myc) (the positive control). The bacterial cells for western blotting were cultured in the presence of 0.2% l -arabinose. All results have been confirmed at least three times. Source data are provided as a Source Data file 6 f Full size image Periplasmic domains of LptF and LptG may transport LPS Our work has showed that both LptF and LptG residues in the cavity of the transporter sf LptB 2 FGC are essential and hydrophobic molecules like detergents can enter via both lateral gates (Supplementary Fig. 8 ). We wondered whether both periplasmic domains of LptF and LptG are crucial for the functionality of the transporter. To test this, we generated single or double mutants located in the core of β-jellyroll-like periplasmic domains of LptF or LptG and performed functional assays. Mutants of conserved residues of W204D, I163D and L206D in LptG and R212E/Y230E, P139D/F149D, Y230E and F149D in LptF are lethal or severely impair cell growth (Fig. 7a–f ). The lethality of I163D may be due to the lowered protein expression compared to that of the wild type. Nevertheless, both periplasmic domains contain functional residues that are crucial for LptB 2 FGC, which might suggest that both of the periplasmic domains of LptF and LptG are involved in LPS transport. Fig. 7 Function of periplasmic domains of LptF and LptG. The structure of the β-jellyroll-like periplasmic domains of LptF and LptG is similar to that of LptC. a Cartoon representation of LptF. Hydrophobic β-jellyroll-like core residues F149, P139, Y230 and R212 are shown in stick. b Functional assays of LptF residues. Residues D129 and E265 are at the neck of the cavity as a control. Mutants R212E/Y230E, P139D/F149D, Y230E and F149D are lethal, while mutants D129A/E265A, R212E and P139D do not have any impact on cell growth. c Protein expression level of the mutants was detected by western blotting. Protein expression levels of other mutants are higher than that of P139D. Source data are provided as a Source Data file (7 c ). d Cartoon representation of LptG. Hydrophobic β-jellyroll-like core residues I163, W204, L206 and V209 are shown in stick. e Functional assays of LptG residues. K62 is located at the cavity as a control, and the mutant K62E grows the same as the wild type. Mutants W204D, I163D, and L206D are lethal, and mutant V209D reduces the cell growth. f Protein expression level of mutants was detected by western blotting. Protein expression level of other mutants is higher than that of mutant K62E except mutant I163D. The lethality of mutant I163D might cause by the lower protein expression. Source data are provided as a Source Data file (7 f ) Full size image The three cryo-EM structures have revealed different conformations of transporter and distinct configurations of the bound LPS in the presence and absence of LptC, which allowed us to speculate the function of LptC in the transporter. In the sf LptB 2 FGC LPS-bound structure, the TM helix of LptC located between TM1G and TM5F opens up the lateral gate and enlarges the central cavity (Fig. 3a–d ). Residues from TM helices of all LptC, LptG and LptF in the cavity make interactions with the bound LPS suggesting all three protein components are involved in LPS binding (Supplementary Fig. 7 ). However, both sf LptB 2 FG and sf LptB 2 FGC structures trapped LPS, suggesting that extracting LPS from the IM into the cavity is not determined by the presence of LptC but LptC is present to facilitate the entry of LPS and direct its transport toward the bridge. Deletion of the full length LptC greatly diminishes LPS transport to LptA [42] , suggesting its importance in bridging the IM transporter and periplasmic protein LptA. Moreover, the enlarged cavity in the sf LptB 2 FGC structure resulted in weaker LPS binding in the cavity with reduced interactions between LPS and cavity residues compared to sf LptB 2 FG (Fig. 2a, b and Supplementary Fig. 7 ), implicating the regulatory role of LptC in making LPS transport more energy efficient. This is also supported by the reduced ATPase activity of sf LptB 2 FGC compared to sf LptB 2 FG under the same conditions (Supplementary Fig. 1 ). The TM helix of LptC opens up the lateral gate TM1G and TM5F, makes a possible entrance for LPS into the cavity supporting the reported models [36] , [37] (Supplementary Figs. 12 and 13 ). On the other hand, one of the LPS acyl tails and an amphipathic detergent molecule interact at the opposite lateral gate (TM1F/TM5G) of the structures, which may suggest that this lateral gate TM1F/TM5G could also be accessible by LPS or amphipathic molecules in cells (Supplementary Fig. 8 ). In the sf LptB 2 FGC structure, LptF makes most of interactions with LptC, and LptG only interacts with LptC through one residue. Two recently reported structures show that the periplasmic domain of LptC connects to that of LptF [36] , [37] , this makes one to recognise the importance of LptF in LPS transport (Supplementary Fig. 13 ). On the other hand, our mutagenic studies reveal that the residues of LptG both in the TM cavity and periplasmic domain show remarkable functional importance to cell viability. Moreover, the trapped LPS molecule in the sf LptB 2 FGC structure shifted 7.3 Å toward LptG compared with the LPS in sf LptB 2 FG structure (Fig. 3e, f ). As a result, we speculate that LptG also has important roles in LPS recognition and transportation. Further investigations are required to clarify the exact path of LPS transported within the transporter system. In the sf LptB 2 FGC AMP-PNP-bound structure, the TM helix of LptC moves away from the LPS-binding cavity. As a result, the TM helices of LptF and LptG may be able to move freely to change conformation to expel LPS out of the cavity. A comparison of the structures shown here provides insight into the transport cycle of sf LptB 2 FGC. In the nucleotide-free state, both the NBDs and TMDs are in open conformations. An LPS in the outer leaflet of the IM binds laterally into the central channel of sf LptB 2 FG through an open lateral gate (Figs. 1c, d and 5c and Supplementary Fig. 8 ). The opening of lateral gates in this state exposes LPS-binding elements in the lumen of the TM channel. Interactions of the hydrophobic and charged residues of the TM helices with the six fatty acyl chains and phosphate groups of LPS may provide sufficient strength and specificity for LPS extraction (Fig. 2a, b ). Upon nucleotides binding, two NBDs dimerise into a closed conformation (Fig. 5a ), triggering conformational changes in the TMDs via the coupling helices and probably the cytoplasmic loop 2. The conformational changes in the NBDs induce an anti-clockwise rotation of the TM helices of LptF and LptG towards the centre to close the cavity (Fig. 5e and Supplementary Movies 1 and 2 ), like the closing motion of a camera lens aperture. The two arginine residues (R292 of LptF and R301 of LptG) identified interacting with the bound nucleotides may have roles in switching the states of the lateral gates of sf LptB 2 FGC as these residues locate on the loop 2 that links respective TM5 of LptF and LptG composing the lateral gates. When comparing the ‘ trans ’ and ‘ cis ’ conformations of TM1 and TM5 of the lateral gates at the two states (Supplementary Fig. 8 ), it is apparent that the gates are in closed states when the complex binds to AMP-PNP (Fig. 5c, d ). The induced inward rotation of the TM helices results tightened TM cavity (Fig. 5a, b ), squeezing the bound LPS into the periplasmic domain of LptB 2 FGC. The structure of the periplasmic domains of LptF and LptG are similar to that of LptC [38] , [39] , and the periplasmic protein LptA shares a common fold with LptC [16] , [18] , [35] , [43] , [44] , [45] and the N terminal domain of LptD [21] , [22] . Together they form a head-to-tail oligomer with a continuous whirling orientated hydrophobic groove bridging between the IM and the OM [25] , [30] , [46] , [47] , [48] . The rotational motion of LptB 2 FGC observed in our structures agrees with the models proposed before [11] , [25] , [46] that the rotating action from the base brings the bound LPS into the spiralling bridge. The design of the rotational mechanism and the need of LptC allows efficient transport of LPS through membrane bridge powered only by LptB 2 FG. The non-hydrolysable nucleotide AMP-PNP binding is able to induce conformational change suggesting that LPS expelling does not require ATP hydrolysis. The arginine residues on the loop 2 interact with the first phosphate group of AMP-PNP suggesting that the conformation of the transporter will only return to the original ‘open’ state when the nucleotide is released after hydrolysis. Our cryo-EM structures of sf LptB 2 FGC show similarities in the TM domains and nucleotide-binding domains of the transporter when superimposed with previously published cryo-EM or crystal structures (Supplementary Fig. 13 ). The periplasmic domains of LptF and LptG are however shown at different conformations, revealing their flexibility. These data suggest that the structure of LptB 2 FGC is highly conserved across species, which makes it an important protein machinery complex to study for understanding the biosynthesis of Gram-negative bacterial membrane. In summary, our cryo-EM structures reveal two important intermediate states of sf LptB 2 FGC at high resolution, providing molecular basis for substrate recognition and ATP induced conformational change of LptB 2 FGC. The comparison of the conformations provides a full picture of the transporting mechanism of LptB 2 FGC at the NBDs and TMDs. This finding confirms rotational transporting model and explains how energy efficiency is achieved by the ABC transporter in the presence of LptC. Expression and purification of LptB 2 FGC and LptB 2 FG Gene fragments containing lptB and lptF-lptG of S. flexneri strain were amplified separately by PCR and subsequently cloned into a pTRC99a plasmid ( Eco RI/ Kpn I restriction digestion for lptB and Kpn I/ Xba I digestion for lptF-lptG ), resulting a pTRC99a- lptB 2 FG construct with an octa-histidine (8 × His) tag at the C terminus of LptB. Primers are listed in Supplementary Table 2 . 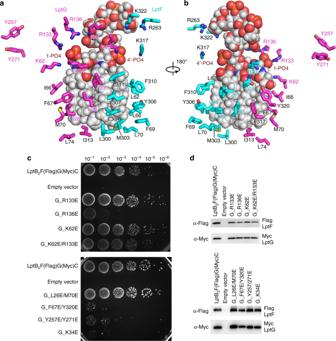Fig. 2 sfLptB2FG recognition of LPS.aResidues of LptF and LptG from the cavity that interact with LPS. LPS is shown in sphere and grey, whereas residues of LptF and LptG are shown in cyan and magenta, respectively.b180° rotation ofaalongy-axis.cFunctional assays of LptG residues. Mutants R136E, F67E/Y320E, Y257E/Y271E and K34E are lethal, whereas mutants R133E, K62E and L26E/M70E do not affect the bacterial growth.dExpression level of LptF and LptG of the mutants. The western blot showed that the mutant protein expression levels are similar to that of the wild type. Source data for paneldare provided as a Source Data file The resulting plasmid was transformed into E. coli C43 (DE3) cells (Novagen) for protein expression. The bacterial cells were grown in Luria broth (LB) supplemented with antibiotic (100 µg ml −1 ampicillin) at 37 °C until the optical density of the culture reached 0.6 at a wavelength of 600 nm (OD 600 ). LptB 2 FG expression was induced with 0.1 mM isopropyl-β- d -thiogalactopyranoside (IPTG) at 20 °C for 6 h. The lptC gene was amplified from S. flexneri strain and the plasmid pTRC99a- lptB 2 FG was linearised by PCR individually. Subsequently, the fragments of lptC and pTRC99a- lptB 2 FG were ligated to create pTRC99a- lptB 2 FGC . C43 (DE3) cells transformed with pTRC99a- lptB 2 FGC were cultured and induced at the same conditions as described above for over-expression of LptB 2 FG. Cultures were harvested by centrifugation and cell pellets were resuspended in purification buffer (20 mM HEPES pH 7.8 and 300 mM NaCl) supplemented with 0.1 mM phenylmethylsulphonyl fluoride (PMSF, Sigma-Aldrich). The cells were lysed by three passes through a cell disrupter (ATS Engineering Ltd) and cell debris was removed by centrifugation at 18,000 × g for 15 min at 4 °C. Membranes were pelleted by ultracentrifugation at 100,000 × g for 1 h at 4 °C and solubilized in purification buffer supplemented with 10 mM imidazole and 1% (w/v) n -dodecyl-β- d -maltopyranoside (DDM) (Anatrace) by stirring at room temperature for 1 h. The suspension of solubilized protein was ultracentrifuged at 100,000 × g for 1 h before being loaded onto a 5 ml HisTrap HP column (GE HealthCare). The column was washed with purification buffer supplemented with 0.05% Lauryl Maltose Neopentyl Glycol (LMNG) and 50 mM imidazole and bound protein was eluted with purification buffer supplemented with 0.05% LMNG and 300 mM imidazole. The protein eluted from Histrap HP column was further purified by size-exclusion chromatography using a Superdex 200 Increase 10/300 column (GE Healthcare) equilibrated in 20 mM HEPES, pH 7.8, 150 mM NaCl and 0.05% LMNG. The purities of the protein fractions were analysed by SDS–PAGE. Fractions with highest purity were collected and concentrated for cryo-sample preparation. For sf LptB 2 FGC AMP-PNP bound, the purified sf LptB 2 FGC was incubated with 5 mM β-γ-imidoadenosine 5′-phosphate (AMP-PNP) and 2 mM MgCl 2 for 1 h at room temperature before cryo-sample preparation. ATPase activity assay ATPase activity assay was performed using ATPase/GTPase Activity Assay Kit (Bioassay Systems). C43 (DE3) cells carrying sf LptB 2 FGC, sf LptB 2 FG or their mutated plasmids were cultured in 1 l LB medium. Cells were induced, collected and lysed using the protocol described above. Solubilised membrane fraction was ultracentrifuged at 100,000 × g for 30 min and the supernatants of each sample were loaded onto a gravity column containing 2 ml pre-balanced Ni 2+ -NTA beads. The columns were washed with 15 column volumes of wash buffer (20 mM HEPES pH 7.8, 300 mM NaCl, 50 mM imidazole and 0.05% LMNG), and eluted with the elution buffer (20 mM HEPES pH 7.8, 300 mM NaCl, 300 mM imidazole and 0.05% LMNG). All samples were further purified using size-exclusion chromatography with a Superdex 200 Increase 10/300 column (GE Healthcare). Protein concentration of the samples was determined using detergent compatible Pierce BCA Protein Assay Kit (Thermo Scientific) according to the manufacture’s instruction. Briefly, 2.5 μl of purified protein was diluted to 25 μl for the BCA assay. The albumin (BSA) was used as the standard. An aliquot of 200 μl of working reagent (made by mixing reagent A and reagent B at 50:1 volume ratio) was added to each sample and incubated at 37 °C for 30 min. Absorbance at 562 nm was measured and the protein concentration of each sample was determined. The ATPase activity assays were carried out in 96-well plates. The phosphate standards and blank control for colorimetric detection was prepared according to the manufacturer’s instructions (ATPase/GTPase Assay Kit, Bioassay systems). An aliquot of 1 μl (1–2 mg ml −1 ) of samples was mixed with 4 μl detergent buffer (20 mM HEPES, pH 7.8, 150 mM NaCl and 0.05% LMNG) and 5 μl assay buffer (ATPase/GTPase Assay Kit) to make 10 μl ATPase activity assay sample. 30 μl reaction solution (made by 20 μl assay buffer plus 10 μl 4 mM ATP solution) was added into each ATPase activity assay sample and incubated at room temperature for 15 min. The reaction was terminated by adding 200 μl reagent (ATPase/GTPase Assay Kit) into each sample and further incubated for 30 min. The absorbance at 600 nm was measured. For AMP-PNP inhibition, sf LptB 2 FGC was incubated with 2 mM AMP-PNP and 5 mM MgCl 2 at 37 °C for 30 min before ATPase activity assay was performed. All assays were repeated six times. ATPase activities of all samples were determined using the mean value of the samples according to the linear regression of standards. All experiments were repeated at least three times. Site-directed mutagenesis and functional assays All single or double mutations were generated following the site-directed mutagenesis protocol published by Liu and Naismith [49] . The functional assays were conducted on the E. coli lptFG chromosomal deletion strain NR1113 (Courtesy to N. Ruiz.) [13] . lptFG deletions are lethal, therefore NR1113 carries a rescue copy of lptFG operon with ampicillin resistance and P BAD promotor, which is inducible by arabinose. The pTRC99a plasmid’s ampicillin resistance gene was replaced by a kanamycin resistance gene, which was then used as the vector for the E. coli LptB 2 FGC mutagenesis. In addition to the His ×8 tag at the C terminus of LptB, we also inserted a Flag tag at residue 138 of LptF (LptF-138-Flag) and a c-Myc tag at 144 of LptG (LptG-144-Myc) to generate the resulting plasmid pTRC99a- E. coli LptBF138G144C -Kan. These single or double mutants were transformed into the E. coli lptFG deletion strain NR1113 [13] . The transformed E. coli cells were grown on LB agar plate supplemented with antibiotics (kanamycin 50 µg ml −1 ) and 0.2% l -arabinose at 37 °C for 12 h. Single colonies of each transformation were inoculated into 10 ml LB medium supplemented with the antibiotics and 0.2% (w/v) l -arabinose. The cells were cultured in an incubator at 200 r.p.m. and at 37 °C for 12 h. Subcultured cells were used for the functional assays. The E. coli NR1113 with the empty plasmid pTRC99a-Kan was used as the negative control, while the NR1113 strain with the plasmid pTRC99a-Kan-LptBF(Flag)G(Myc)C or the NR1113 strain in the presence of 0.2% l -arabinose was used as the positive control. Cell pellets were harvested, washed twice and diluted in sterile LB medium to the OD 600 nm of 0.5. Tenfold serial dilution functional assays were performed. The dilution range was from 10 −1 to 10 −6 and 5 µl of the diluted cells was dripped onto the LB agar plates containing kanamycin 50 μg ml −1 . Cell growth was observed after overnight culture at 37 °C. All the assays were performed in triplicate. Western blotting The protein expression of the LptFG mutants were determined by western blotting. An aliquot 0.5 ml of overnight cultures of transformed NR1113 cells with LptB 2 FGC or mutants was inoculated into 50 ml LB supplemented with antibiotics (kanamycin 50 µg ml −1 ) and 0.2% l -arabinose. The cells were cultured at 37 °C for 6 h and harvested by centrifugation. The cells were resuspended in 1 ml buffer containing 20 mM Tris-Cl, pH 7.8 and 150 mM NaCl supplemented with 1 mM PMSF. The cells were lysed by sonication for 1 min on ice. The membrane fraction was harvested and solubilized with 1% DDM for 20 min at room temperature. The undissolved debris was removed by centrifugation at 13,000 × g for 10 min at 4 °C. The supernatant was loaded to a Ni 2+ -NTA column and washed with a buffer containing 0.05% DDM, 20 mM Tris-Cl pH 7.8, 150 mM NaCl and 30 mM imidazole. The protein was eluted with 0.05% DDM, 20 mM Tris-Cl pH 7.8, 150 mM NaCl and 500 mM imidazole. The eluted samples were mixed with 4 × SDS–PAGE loading buffer and incubated at 98 °C for 10 min. The samples were centrifuged at 13,000 × g for 1 min, and 10 μl of each sample was loaded onto 12% Bis-Tris Plus SDS–PAGE gel for the immunoblot analysis. The proteins were transferred to a PVDF membrane using the Mini Transfer-Blot (Bio-Rad) at 100 V for 1 h. The PVDF membranes were blocked in 1× phosphate buffered saline Tween-20 (PBST) supplemented with 5% skim milk at 4 °C for 1 h. The membranes were incubated with anti-Flag (Sigma, Catalogue No: F3165) or anti-Myc monoclonal antibody (1:300 dilution) (Sigma, Catalogue No: A5963) at room temperature for 1 h. The membranes were washed with PBST four times and then incubated with rabbit anti-mouse IgG antibody (1:5000 dilution) for 1 h. The membranes were washed with PBST four times and PBS twice. Protein bands were visualised by chemiluminescent in a photo imager (Bio-Rad). Sample preparation and cryo-EM data acquisition 2.5 μl of purified protein complex at a concentration of ~1 mg ml −1 was applied to glow-discharged Quantifoil holey carbon grids (R1.2/1.3, 300 mesh, copper). Grids were blotted for 3.5 s with the environmental chamber set at 95% humidity and flash-frozen in liquid ethane cooled by liquid nitrogen using Vitrobot Mark IV (FEI). Grids were imaged with a Titan Krios (FEI) electron microscope, operated at 300 keV equipped with a K2 Summit electron counting direct detection camera (Gatan). Datasets were collected in super-resolution mode using the automated data collection programme SerialEM [50] . All cryo-EM images were recorded in super-resolution mode and images were acquired at a nominal magnification of ×29,000, corresponding to a calibrated physical pixel size of 1.014 Å. Defocus range was set between −1.5 and −2.5 μm. Each image was acquired at an exposure time of 8 s and dose-fractionated to 40 frames with a dose rate of about 7 counts per second per physical pixel. Image processing For the cryo-EM data of sf LptB 2 FG LPS bound, the beam-induced motion correction of image stacks were performed using MotionCor2 to generate 2x binned average micrographs and dose-weighted micrographs with a pixel size of 1.014 Å [51] . The contrast transfer function parameters of these average micrographs were estimated by Gctf [52] . Other procedures of data processing were performed in RELION [53] . 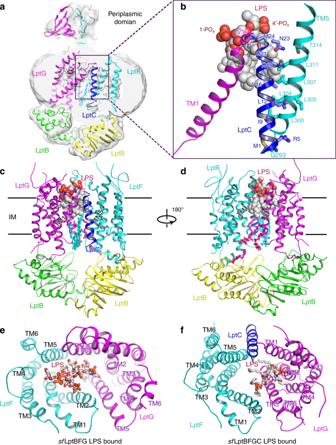Fig. 3 Cryo-EM structure of LPS-boundsfLptB2FGC.aCryo-EM map of LPS-boundsfLptB2FGC. The colour scheme is the same as in Fig.1. LptC is coloured in blue.bA close view of LPS. Lipid A of LPS is visible in the complex and LptC transmembrane helix is at the lateral gate TM1G/TM5F. LPS is shown in spheres.cCartoon representation of LPS-boundsfLptB2FGC.dRotation of 180° along they-axis relative toc.ePeriplasmic view of LPS-boundsfLptB2FG, where LPS is closed to the LptF side.fPeriplasmic view of LPS-bound sfLptB2FGC. LPS is closed to the LptG side 1,524,391 particles were automatically selected, and finally 95,887 particles were selected for 3D refinement and a reported 3.7 Å resolution map was generated after post-processing with a B -factor of −107 Å 2 . The data processing details are summarised in Supplementary Fig. 2 . The data processing procedures of sf LptB 2 FGC LPS bound were similar to the procedures of sf LptB 2 FG-LPS bound. 1,928,889 particles were automatically selected, and then two-dimensional (2D) and three-dimensional (3D) classifications were performed to select consistent particle classes. Finally, 546,301 particles were selected for 3D refinement and a reported 3.1 Å resolution map was generated after post-processing with a B -factor of −132 Å 2 . The data processing details are summarised in Supplementary Fig. 5 . The data processing procedures of sf LptB 2 FG AMP-PNP bound were similar to the procedures of sf LptB 2 FG-LPS bound. 1,762,877 particles were automatically selected, and then 2D and 3D classifications were performed to select consistent particle classes. Finally, 149,178 particles were selected for 3D refinement and a reported 3.2 Å resolution map was generated after post-processing with a B -factor of −132 Å 2 . The data processing details are summarised in Supplementary Fig. 9 . Model building and refinement Crystal structure of LptB 2 FG of K. pneumoniae (PDB code: 5L75) was fitted into the cryo-EM map of sf LptB 2 FG LPS bound at 3.7 Å, using UCSF Chimera [54] . The model was then built using COOT [55] . The high-resolution cryo-EM maps allow the side chain assignments according to the bulk side chains. There is a very clear map density in the central cavity of sf LptB 2 FG for a rough LPS molecule (Supplementary Figs. 2 and 3 ). An LPS molecule was built in the density using the Ra-LPS model (PDB:3FXI) [56] . There are densities for detergents near the lateral gates, and two LMNG and four DDM molecules are built in sf LptB 2 FG LPS-bound model. Although there are clear densities for the periplasmic domains of LptF and LptG, the periplasmic domains were not able to be built due to the low resolution. 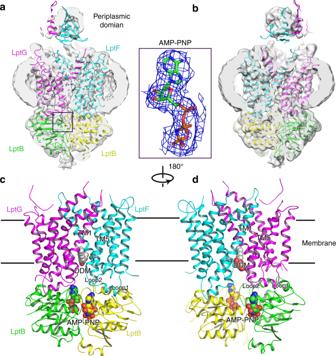Fig. 4 Structure of AMP-PNP-boundsfLptB2FGC.aCryo-EM map of AMP-PNP-boundsfLptB2FGC. The LptC density is not observed. Density of AMP-PNP is shown in blue mesh and AMP-PNP is shown in stick. The colour scheme is the same as Fig.1.bRotation of 180° along they-axis relative toa.cCartoon representation of AMP-PNP-boundsfLptB2FGC. AMP-PNP is shown in spheres with carbon colour in green or yellow. DDM is shown in sphere with carbon in grey.dRotation of 180° alongy-axis relative toc. The DDM molecule is trapped in the lateral gate TM1F/TM5G The model of sf LptB 2 FG-LPS bound was fitted into the 3.1 Å resolution density map of sf LptB 2 FGC-LPS. There are densities for LptC TM helix, located between the lateral gate TM1G/TM5F, and LPS located in the cavity. Contrast to the LPS trapped in the sf LptB 2 FG, there is no density for the core oligosaccharide of LPS in the sf LptB 2 FGC complex, suggesting the core oligosaccharide is flexible (Supplementary Fig. 6 ). The side chains of sf LptB 2 FGC complex are assigned based on the high-resolution cryo-EM density. There is clear density for the periplasmic domains of LptF and LptG and the two domains are fitted well in the density. The density of the periplasmic domain of LptC is not very clear, suggesting that the periplasmic domain is flexible. Detergent molecules (DDM, LMNG) were built near the lateral gates, where LMNG molecule is trapped in the lateral gate TM1G/TM5F (Supplementary Fig. 8 ). The Crystal structure of LptB 2 FG of K. pneumonia (PDB code: 5L75) is fitted in the density of cryo-EM sf LptB 2 FGC-AMP-PNP bound map at 3.2 Å. The side chains of sf LptB 2 FGC-AMP-PNP bound are assigned based on the high-resolution cryo-EM map, while there is density for the periplasmic domains of LptF and LptG. The TM helix of LptC is no longer at the lateral gate TM1G/TM5F and there is no clear density for LptC periplasmic domain, suggesting that LptC is flexible. The cryo-EM map of sf LptB 2 FGC AMP-PNP bound has two clear densities at the active site of LptB (Fig. 4a–d ) for two AMP-PNP molecules. 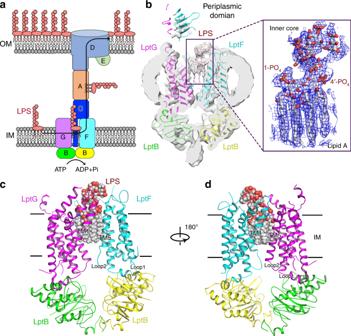There is a density in the cavity through the lateral gate TM1F/TM5G, which we identified it as a DDM molecule (Supplementary Fig. 8 ). 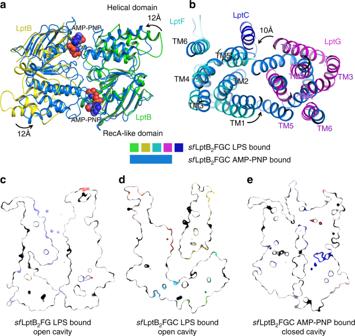Fig. 5 Superimpositions of AMP-PNP and LPS-boundsfLptB2FGC structures.aAMP-PNP binding induces the conformational changes of LptB (NDBs). The helical domains of the dimeric LptB (AMP-PNP-boundsfLptB2FGC) showed a rotational shift of ~12 Å in the anti-clockwise direction from the nucleotide-free state of dimeric LptB (LPS-boundsfLptB2FGC). The LPS-boundsfLptB2FGC is coloured in the same as Fig.1. The AMP-PNP-boundsfLptB2FGC is coloured in marine blue and AMP-PNP shows as spheres.bA top view of superimposed transmembrane helices of LPS-boundsfLptB2FGC and AMP-PNP-boundsfLptB2FGC complex. AMP-PNP binding induces the TM helices of AMP-PNP-boundsfLptB2FGC to rotate in the anti-clockwise direction with the largest shift of ~10 Å from the nucleotide-free state (LPS-boundsfLptB2FGC) towards the central channel.cSlab view of surface representation of cavity of LPS-boundsfLptB2FG. The cavity is in an outward open conformation.dSlab view of cavity of LPS-boundsfLptB2FGC. The cavity is in an outward open conformation. The transmembrane helix of LptC is located at the lateral gate TM1G/TM5F, enlarging the cavity. The neck of the cavity is widely open.eSlab view of cavity of AMP-PNP-boundsfLptB2FGC. The cavity is closed, which is induced by AMP-PNP binding 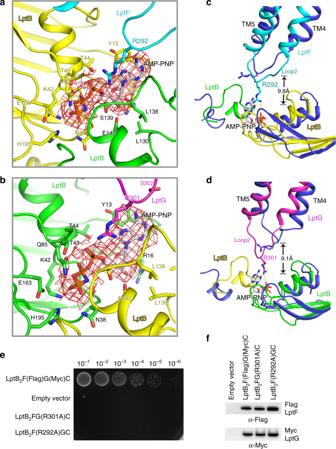Fig. 6 R292 of LptF and R301 of LptG are involved in AMP-PNP binding.aA close view of AMP-PNP binding residues with dimeric LptB and R292 of LptF.bA close view of AMP-PNP binding residues with dimeric LptB and R301 of LptG. AMP-PNP molecules are shown in stick, and the cryo-EM map for AMP-PNP are shown in red mesh.cThe two cryo-EM structures are superimposed. The arginine residue R292 located on the cytoplasmic loop 2 of LptF shifts around 9.8 Å to interact with AMP-PNP.dThe arginine R301 located on the cytoplasmic loop 2 of LptG shifts around 9.1 Å to interact with the AMP-PNP. AMP-PNP molecules are shown in stick, the colour scheme ofsfLptB2FGC AMP-PNP bound is the same as in Fig.4, andsfLptB2FG LPS bound is coloured in blue.eFunctional assays of the single mutants R292 of LptF and R301 of LptG. NR1113 cells were transformed with empty vector (pTRC99a_Kan, the negative control) or the vector encoding LptB2F(Flag)G(Myc)C (the positive control).fDetection of protein expression levels of mutants by western blotting. Empty vector (pTRC99a_Kan, the negative control) or the vector encoding LptB2F(Flag)G(Myc) (the positive control). The bacterial cells for western blotting were cultured in the presence of 0.2%l-arabinose. All results have been confirmed at least three times. Source data are provided as a Source Data file 6f 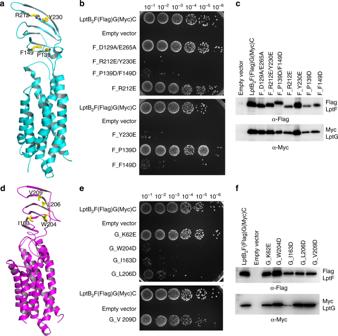Fig. 7 Function of periplasmic domains of LptF and LptG. The structure of the β-jellyroll-like periplasmic domains of LptF and LptG is similar to that of LptC.aCartoon representation of LptF. Hydrophobic β-jellyroll-like core residues F149, P139, Y230 and R212 are shown in stick.bFunctional assays of LptF residues. Residues D129 and E265 are at the neck of the cavity as a control. Mutants R212E/Y230E, P139D/F149D, Y230E and F149D are lethal, while mutants D129A/E265A, R212E and P139D do not have any impact on cell growth.cProtein expression level of the mutants was detected by western blotting. Protein expression levels of other mutants are higher than that of P139D. Source data are provided as a Source Data file (7c).dCartoon representation of LptG. Hydrophobic β-jellyroll-like core residues I163, W204, L206 and V209 are shown in stick.eFunctional assays of LptG residues. K62 is located at the cavity as a control, and the mutant K62E grows the same as the wild type. Mutants W204D, I163D, and L206D are lethal, and mutant V209D reduces the cell growth.fProtein expression level of mutants was detected by western blotting. Protein expression level of other mutants is higher than that of mutant K62E except mutant I163D. The lethality of mutant I163D might cause by the lower protein expression. Source data are provided as a Source Data file (7f) The three structures, sf LptB 2 FG LPS bound, sf LptB 2 FGC LPS bound and sf LptB 2 FGC AMP-PNP bound, were refined using the phenix.real_space_refine in PHINEX [57] . Fig. 1 Architecture of LPS-boundsfLptB2FG complex.aA scheme of seven lipopolysaccharide transport proteins form atrans-envelope bridge to transport LPS from the IM to the OM.bLeft panel: a cross-sectional view of cryo-EM map of LPS-boundsfLptB2FG; Right panel: a closed view of LPS. A clear density for LPS is shown in blue mesh and LPS is shown in stick. LptF, LptG and the two LptB molecules are presented in cartoon and coloured in cyan, purple, green and yellow, respectively.cCartoon representation of LPS-boundsfLptB2FG. An LPS molecule, shown in spheres, is located in the upper cavity of the transmembrane channel.dRotation of 180° along they-axis relative toc Statistics of 3D reconstruction and model refinement can be found in Supplementary Table 1 . Reporting summary Further information on research design is available in the Nature Research Reporting Summary linked to this article.